Sorting of small infectious virus particles by flow virometry reveals distinct infectivity profiles The nature and concentration of lipids and proteins at the surface of viruses are essential parameters for determining particle infectiveness. Historically, averaged bulk analysis of viral particles has been the primary method to quantitatively investigate these parameters, though this neglects heterogeneity within populations. Here we analyse the properties of Junin virus particles using a sensitive flow virometry assay and further sort virions while conserving their infectiveness. This method allows us to characterize the relationship between infectivity, virus size and RNA content and to compare particles secreted by Vero cells with those from physiologically relevant human primary macrophages. Our study highlights significant differences in particle infectivity according to its nature, the type of producer cells and the lipid membrane composition at the budding site. Together, our results present the flow virometry assay as a powerful and versatile tool to define virus particle profiles. The characterization of individual cells within a total population has been within reach since the introduction of flow cytometry decades ago. Additional technology improvements have given researchers the ability to sort populations of interest, cell by cell, with high accuracy while preserving cell viability and allowing further functional assays. Today, the limits of flow cytometry are repeatedly tested by the research community who aims to quantitatively analyse small biological vesicles in a similar way as has been done for cells. However, one of the main limitations of this approach is the low size sensitivity of the cytometry instrumentation, which currently remains around 300 nm at best for conventional cytometers. Lipid bilayer membrane vesicles smaller than 300 nm are numerous both inside and outside the cell, including clathrin-coated vesicles, exosomes and viruses. A few groups have attempted to detect small vesicles by flow cytometry [1] , [2] , [3] , [4] , [5] , [6] , [7] , [8] and one group has sorted fixed bacteriophage particles and sequenced them [8] . Detection of small vesicles is usually performed on non-conventional custom-made cytometers and requires advanced expertise to achieve high-resolution flow cytometry. To the best of our knowledge, no one has succeeded to sort small vesicles while preserving their biological activity. As of today, while cytometry technology continues to improve, this remains a significantly challenging issue. In our study, we use the Junin virus (JUNV) as a model system to explore small vesicle detection, sorting and functionality. JUNV is an enveloped virus and a member of the New World Arenaviridae family. The virus is the causative agent of the Argentine Haemorrhagic Fever, which has high mortality rates in humans (up to 30% fatality of infected patients). Candid1 , an attenuated strain of JUNV, has been shown to confer a high rate of protection against the disease and is used as a live-attenuated vaccine in endemic regions [9] . This strain Candid1 is also widely used as a laboratory model to study the biology of New World Arenaviruses. The genetic material of JUNV is composed of a Short and a Large segment of ambisense single-stranded RNA. Its envelope is a glycoprotein (GPC) responsible for the recognition of the human transferrin receptor at the surface of target cells [10] . Transferrin receptor expression is known to be important for efficient infection and replication of JUNV in cells, although other receptors may also play a role [11] , [12] , [13] . It is well established that the genetic material of RNA virus populations is very heterogeneous. However, heterogeneity of the lipid and protein composition of individual virus particles remain poorly studied, and direct correlation between viral particle content and infectiveness has not been addressed, mainly due to the fact that reliable and sensitive methods have not previously been available. Here we develop and apply advanced flow cytometry techniques to define the infectivity profiles of viral particles according to their composition. We have optimized a very sensitive cytometry-based technique referred to as ‘flow virometry assay (FVA)’ that enables viral particle analysis and sorting, with retention of infectivity of the sorted viruses. The instrument used contains powerful lasers, a digital focusing system (DFS) and advanced optics that enable sorting on the basis of light scattering parameters in combination with fluorescent channels. Here FVA is used to demonstrate that virion size and the envelope GPC concentration at its surface correlates with JUNV infectivity. Moreover, by co-labelling GPC and nucleic acids of viral particles, we determine the proportions of competent particles (RNA + GPC + ) in virus populations, which vary according to the fraction studied. We also compare the ability of Vero cells and human primary macrophages to secrete infectious particles and highlight that infected macrophages produce a vast number of defective particles. Finally, we show that virus particles incorporate lipid microdomain markers such as the tetraspanin CD9 and are positive for the lipid raft marker Cholera toxin B (CTB), and that disruption of these microdomains impairs viral infectivity. In conclusion, this study presents a powerful tool to analyse and sort lipid microvesicles and gives new insights into the biology of the JUNV. Flow cytometry analysis of small particles Along this study, we used a customized version of the commercial FACSAria II Special Order (SORP) cell sorter (BD Biosciences) with a powerful 300 mW 488 nm laser and a DFS option. The instrument was equipped with a photomultiplier tube option for the forward scatter channel (FSC-PMT). The cytometer tubing was extensively cleaned and the flow sheath was highly filtered (0.45 and 0.1 μm filters). The pressure was allowed to stabilize for at least 2 h before starting experiments. First, we tested the sensitivity and resolution of our instrument using various DFS parameters ( Supplementary Fig. 1 ). The DFS is a picomotor-driven focusing device that adjusts the dimension of the beam at its intersection with the core stream to obtain a smaller focal spot resulting in a smaller observation volume, which in turn increases the scatter signal and decreases the background. Optimization of the DFS parameters shows improved capacity of our instrument to discriminate small beads according to their size ( Supplementary Fig. 1 ). Next we investigated whether our instrument could detect fluorescent beads of 40 and 100 nm using FSC-PMT levels and fluorescence intensity in combination ( Fig. 1a–d ). We could detect and discriminate fluorescent latex beads of 40 nm (coupled to APC; Fig. 1a ) and 100 nm (coupled to PE; Fig. 1d ) when the fluorescent channel is also used to trigger detection. However, the beads remained at the level of the background in the FSC-PMT channel. Therefore, only the combination of both fluorescence and reliable FSC-PMT channels allowed higher detection efficiency of nanosized objects, in agreement with previous observations [14] . The 40 nm beads coupled to APC could not be detected with the PE optical band-pass filter (575/25) and the 100 nm beads coupled to PE could not be detected with APC optical bandpass filter ( Fig. 1b,c ). 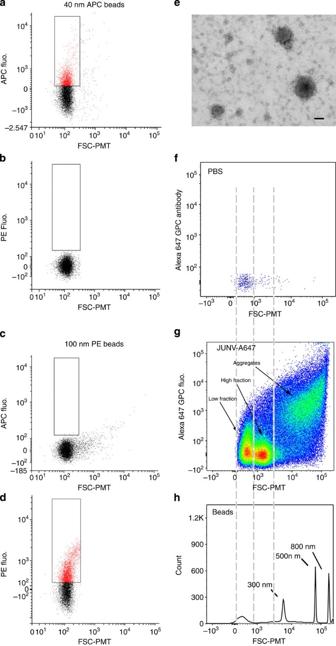Figure 1: Flow cytometry analysis of small particles. (a–d) 40 nm APC-conjugated latex beads (a,b) and 100 nm PE-conjugated latex beads (c,d) were analysed on our custom-made flow cytometer and plotted for APC fluorescence (a,c) or PE fluorescence (b,d) as a function of the FSC-PMT parameter. The 40 and 100 nm beads were specifically detected from their respective fluorophores. (e) JUNVs concentrated by ultracentrifugation were adsorbed on carbon-coated EM grids and labelled with the GPC-specific LD05 mouse monoclonal antibody followed by a secondary anti-mouse antibody and revealed by Protein A 10 nm gold beads. Contrast was obtained by negative staining. Scale bar, 50 nm. JUNV particles of various sizes were all positive for the GPC antibody staining. (f,g) Flow virometry analysis of PBS (f) or purified viral particles stained with a GPC antibody coupled to an Alexa Fluor 647 (JUNV-A647;g). The plot shows Alexa 647 GPC fluorescence versus FSC-PMT. Both samples were run using the same parameters, at the same speed and for the same amount of time. (g) Several populations could be distinguished and are pointed out by labelled arrows. Fluorescence-based thresholding was used to decrease noise events. (h) Non-fluorescent polystyrene beads of larger size (300, 500 and 800 nm) were detected by FSC-PMT channel only. The area between the two first grey dashed lines shows FSC-PMT events that are at the level of the background. The area between the second and third dashed lines correspond to events above background but smaller than 300 nm. Figure 1: Flow cytometry analysis of small particles. ( a – d ) 40 nm APC-conjugated latex beads ( a , b ) and 100 nm PE-conjugated latex beads ( c , d ) were analysed on our custom-made flow cytometer and plotted for APC fluorescence ( a , c ) or PE fluorescence ( b , d ) as a function of the FSC-PMT parameter. The 40 and 100 nm beads were specifically detected from their respective fluorophores. ( e ) JUNVs concentrated by ultracentrifugation were adsorbed on carbon-coated EM grids and labelled with the GPC-specific LD05 mouse monoclonal antibody followed by a secondary anti-mouse antibody and revealed by Protein A 10 nm gold beads. Contrast was obtained by negative staining. Scale bar, 50 nm. JUNV particles of various sizes were all positive for the GPC antibody staining. ( f , g ) Flow virometry analysis of PBS ( f ) or purified viral particles stained with a GPC antibody coupled to an Alexa Fluor 647 (JUNV-A647; g ). The plot shows Alexa 647 GPC fluorescence versus FSC-PMT. Both samples were run using the same parameters, at the same speed and for the same amount of time. ( g ) Several populations could be distinguished and are pointed out by labelled arrows. Fluorescence-based thresholding was used to decrease noise events. ( h ) Non-fluorescent polystyrene beads of larger size (300, 500 and 800 nm) were detected by FSC-PMT channel only. The area between the two first grey dashed lines shows FSC-PMT events that are at the level of the background. The area between the second and third dashed lines correspond to events above background but smaller than 300 nm. Full size image The 100-nm beads coupled to PE are at the limit of detection of the PMT-forward scatter alone. A main population (>95%) is found at the level of the noise, while few doublets (200 nm) and higher aggregates can also be detected ( Supplementary Fig. 2a ). Some of the events detected at the level of the noise have a low but significant fluorescent intensity ( Supplementary Fig. 2b ), suggesting that they are individual beads. Doublets can be detected by FSC-PMT alone but further confirmed when correlated by the higher fluorescence intensity ( Supplementary Fig. 2c ). In conclusion, our flow cytometer allows detection of 40 and 100 nm objects by combining FSC-PMT and fluorescence intensity. FVA of the JUNV Arenaviruses are quite heterogeneous in size as represented in Fig. 1e . The JUNV particle ranges from 40 to 250 nm (ref. 15 ) and is thus a good model to evaluate the ability of our system to detect small vesicles. Since cytometry refers to the measurement of cells, we call our method FVA, to refer to the measurement of viruses [7] . JUNV particles were labelled with the Alexa Fluor 647-conjugated antibody LD05 that specifically recognizes the envelope GPC of JUNV ( Fig. 1e ). This antibody has the advantage of being non-neutralizing ( Supplementary Fig. 3a and ref. 16 ) and can therefore be used in infectivity assays. This preparation of Alexa Fluor 647-labelled JUNV particles (JUNV-A647; see Methods) was analysed by FVA, where at least ten thousands of events were recorded ( Fig. 1g ). At the same flow rate and time of analysis, running PBS alone (filtered with 0.1 μm filter) leads to very limited background signal in both FSC-PMT and fluorescent channels and very few events could be recorded ( Fig. 1f ). Two JUNV-A647 positive populations, which we will refer to as the low and high fractions, were distinctly discriminated by size using the FSC-PMT channel in combination with fluorescence intensity using the 640 nm laser channel ( Fig. 1g ). A third population, most likely corresponding to viral aggregates, was observed. Using the same parameters, comparison of polystyrene beads ( Fig. 1h ) and JUNV-A647 preparations ( Fig. 1g ) suggests that the virus particles contained in the low and high fractions are smaller than 300 nm, as expected for Arenaviruses (personal observations and ref. 15 ). The particles present in the low fraction have a FSC-PMT at the level of the noise, but the fluorescent channel is above background (as for the 40 nm APC beads) and allows discriminating them from background (see gating in Supplementary Fig. 3b ). Of note, JUNV particles are at least as bright as 40 nm APC beads ( Supplementary Fig. 3c,d ), therefore confirming that FVA is sensitive enough to detect very small viral particles that FSC-PMT could not resolve alone. Sorting of JUNV particles The relationship between size and scatter parameters of polystyrene beads and lipidic vesicles is not straightforward due to their different refractory indexes, and also depends on the laser alignment and optical configuration of the instrument used [17] . To more accurately estimate the size of virus particles in each fraction, JUNV particles analysed by FVA were further sorted onto negatively charged carbon-coated grids maintained in position by a custom-made holder that allows overflow to be evacuated while viruses adsorb on the grid surface. After the low and high fractions were sorted onto these grids, the particles were labelled with a GPC-specific antibody revealed by Protein A coupled to 10 nm gold beads and negatively stained (see Methods) for transmission electron microscopy (EM) imaging. We consistently observed viral particles of ≈60 nm from the low fraction ( Fig. 2a ) and of ≈150 nm from the high fraction ( Fig. 2b ). We observed minimal side-to-side or aggregated viruses in these fractions. At this stage, precise size quantification remain difficult as some virions were damaged, likely due to particles hitting the grid at high speed and the strong chemical treatments of EM processing. To further confirm our ability to sort viral particles smaller than 300 nm, we ran sorted particles through the qViro-X Izon tunable resistive pulse sensing (TRPS) system. TRPS is a relatively recent technique used for high-throughput individual nanoparticle resolution measurements as particles are driven through a size-tunable nanopore (see Methods and ref. 18 for details). Unsorted JUNV particles show a wide size distribution ( Fig. 2c , blue bars), while sorted particles gated on A647 fluorescent particles with FSC-PMT below 300 nm present a smaller mean size with >95% particles indeed below 300 nm (pink bars). Of note, we could not detect particles below 90 nm in the settings used. 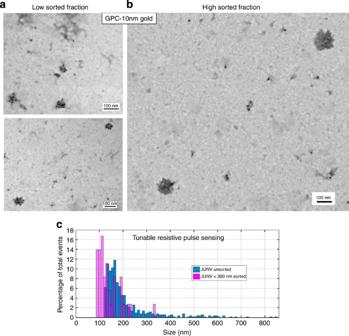Figure 2: Sorting of infectious viruses by flow virometry. (a,b) JUNV-A647 particles were sorted directly onto carbon-coated EM grids and labelled with the GPC-specific GD01 antibody followed by a secondary antibody and then revealed by Protein A 10 nm gold beads. The low (a) and high (b) fractions were negatively stained and analysed by transmission electron microscopy. Several particles per micrograph are shown and the images are representative of each population. The low fraction viruses are about 60 nm in diameter, while the high fraction viruses are around 150 nm. (c) TRPS was performed on unsorted (blue bars) or sorted particles smaller than 300 nm (pink bars). The histograms show the distribution of particle size detected in each sample. Figure 2: Sorting of infectious viruses by flow virometry. ( a , b ) JUNV-A647 particles were sorted directly onto carbon-coated EM grids and labelled with the GPC-specific GD01 antibody followed by a secondary antibody and then revealed by Protein A 10 nm gold beads. The low ( a ) and high ( b ) fractions were negatively stained and analysed by transmission electron microscopy. Several particles per micrograph are shown and the images are representative of each population. The low fraction viruses are about 60 nm in diameter, while the high fraction viruses are around 150 nm. ( c ) TRPS was performed on unsorted (blue bars) or sorted particles smaller than 300 nm (pink bars). The histograms show the distribution of particle size detected in each sample. Full size image Infectivity profiles of sorted particles Taking advantage of our ability to sort viruses, we investigated whether viral particles were still infectious post sort, and if so, what the infectious properties of the low and high fractions were. Infectiveness of 3,000 viral particles sorted from the low and high populations was evaluated by plaque assay ( Fig. 3a ). We reproducibly observed a twofold increase of infectivity from the high fraction compared with the low fraction ( Fig. 3b ). As the viruses from the high fraction could contain more genomic RNA (explaining their increased infectivity), we quantified the amount of short and large RNA segments by reverse transcription real-time quantitative PCR (RT-qPCR) from 20,000 sorted viruses from each fraction. At equal particle number, the high and the low fractions contain similar amounts of both short and large RNA segments ( Fig. 3c ), suggesting that the increased infectivity of the particles from the high fraction is independent of their viral RNA content. Moreover, the ratio between the short and the large RNA segments of JUNV was similar in both fractions as well as the unsorted JUNV stock ( Fig. 3d ), further indicating that sorted virus fractions share similar genomic properties. 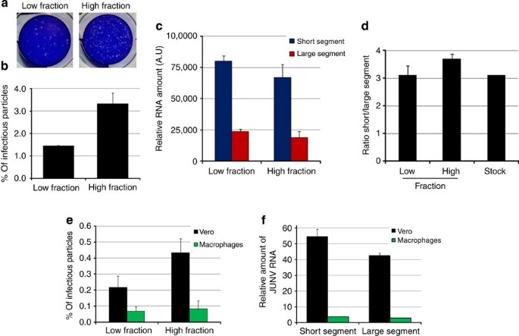Figure 3: Infectious properties of sorted particles from the low and high fractions. (a,b) Confluent Vero cells were infected with 3,000 sorted particles in 300 μl virus media for 1 h, subsequently overlaid with virus media containing 1% melted agarose and incubated for 5 days. Plaques forming units were revealed by crystal violet staining. (a) Images correspond to plaques observed in representative wells infected with 3,000 particles from the low (left) and high (right) fractions. (b) Quantification of the percentage of infectious particles from the low and high fractions. Error bars are mean±s.d. of duplicates and the histogram is representative of four independent experiments. (c) Relative amount of RNA contained in 20,000 sorted particles for each fraction. Reverse transcriptase RT-qPCR with primers targeting the short (blue) or the large (red) segment of JUNV is shown. Low and high fractions showed similar RNA levels for both short and large segments. Error bars are the mean±s.d. of triplicates and the data are representative of two independent experiments. (d) Ratio of the relative amount of short to large segment in the low and high fractions and in the virus stock. RNA ratio remains constant in all three samples. (e) Quantification of the percentage of infectious particles produced by Vero cells (black bars) or human primary macrophages (green bars) from the low and high fractions. (f) Relative amount of RNA contained in 15,000 sorted particles from Vero cells (black bars) or human primary macrophages (green bars). Reverse transcriptase RT-qPCR with primers targeting the short or the large segment of JUNV is shown. Error bars are the mean±s.d. of triplicates. Figure 3: Infectious properties of sorted particles from the low and high fractions. ( a , b ) Confluent Vero cells were infected with 3,000 sorted particles in 300 μl virus media for 1 h, subsequently overlaid with virus media containing 1% melted agarose and incubated for 5 days. Plaques forming units were revealed by crystal violet staining. ( a ) Images correspond to plaques observed in representative wells infected with 3,000 particles from the low (left) and high (right) fractions. ( b ) Quantification of the percentage of infectious particles from the low and high fractions. Error bars are mean±s.d. of duplicates and the histogram is representative of four independent experiments. ( c ) Relative amount of RNA contained in 20,000 sorted particles for each fraction. Reverse transcriptase RT-qPCR with primers targeting the short (blue) or the large (red) segment of JUNV is shown. Low and high fractions showed similar RNA levels for both short and large segments. Error bars are the mean±s.d. of triplicates and the data are representative of two independent experiments. ( d ) Ratio of the relative amount of short to large segment in the low and high fractions and in the virus stock. RNA ratio remains constant in all three samples. ( e ) Quantification of the percentage of infectious particles produced by Vero cells (black bars) or human primary macrophages (green bars) from the low and high fractions. ( f ) Relative amount of RNA contained in 15,000 sorted particles from Vero cells (black bars) or human primary macrophages (green bars). Reverse transcriptase RT-qPCR with primers targeting the short or the large segment of JUNV is shown. Error bars are the mean±s.d. of triplicates. Full size image The content of viruses released may differ according to the producer cell type. Thus, we compared JUNV particles produced by the widely used Vero cell line or by primary human macrophages derived from purified monocytes from healthy blood donor (see Methods for details). Macrophages or Vero cells infected for 1 h with JUNV (multiplicity of infection 1) were extensively washed and incubated for 36 h at 37 °C and 5% CO 2 . The supernatant was processed as in Fig. 1g . On sorting, infectivity assays performed by plaque assays revealed that JUNV particles produced by macrophages are poorly infectious compared with Vero-produced JUNV particles, regardless of their size ( Fig. 3e ). Moreover, at same particle number, macrophages-derived JUNV presents a 10-fold decrease in RNA content when compared with Vero-derived JUNV ( Fig. 3f ), which could explain their poor infectivity efficiency. Correlation between GPC levels and RNA content Since analysis of virus populations by RT-qPCR may misrepresent the actual distribution of RNA in viral particles, we took advantage of our FVA to analyse GPC expression and RNA content of the JUNV particles. Labelling of virions with either a GPC antibody ( Fig. 4a ) or with the high affinity nucleic acid dye YOYO-1 ( Fig. 4b ) highlighted that no crosstalk between channels occurs. Of note, JUNV particles contain ribosomes and we cannot exclude that the YOYO-1 staining detected by FVA represents a contribution from both ribosomal and genomic RNAs. Co-labelling of GPC and nucleic acids for analysis by FVA ( Fig. 4c ) allowed us to determine the amount of GPC + RNA + particles within the population, with these corresponding to the pool of likely infectious particles as they contains two elements indispensable for virus infectivity. Interestingly, while the percentage of total RNA + particles (GPC + and GPC − ) is similar in both fractions ( Fig. 4d , green slices), the high fraction contained 2.5 times more RNA + GPC + particles than the low fraction ( Fig. 4d , yellow slices). This finding could thus explain the increase in infectivity of the high fraction observed in Fig. 3b . RT-qPCR of 20,000 particles from total RNA + or GPC + RNA + viral particles revealed that the GPC + RNA + particles are enriched in JUNV RNA ( Fig. 4e,f ), further indicating that these particles correspond to the pool of potentially infectious viruses. 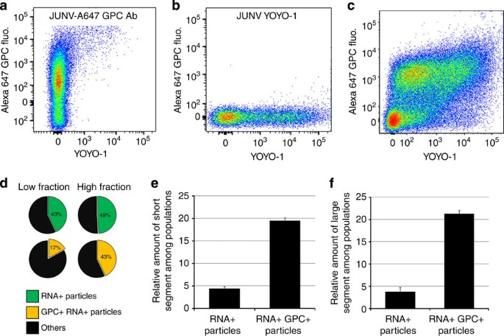Figure 4: Correlation between GPC levels and RNA content. FVA of JUNV particles stained with Alexa 647 GPC antibody only (a) or YOYO-1 only (b). Dot plots represent nucleic acid dye fluorescence (xaxis) as a function of the Alexa 647 GPC fluorescence (yaxis). (c) Flow virometry analysis of particles stained with both Alexa 647 GPC antibody and the nucleic acid dye YOYO-1. (d) Pie charts representing the percentage of total RNA+ vesicles (green) and the percentage of potentially infectious particles (GPC+RNA+; yellow) in the low and high fractions. The high fraction contains about 2.5 times more virions with both genetic material and surface GPC than the low fraction. (e,f) Relative amount of RNA contained in 20,000 sorted particles from total RNA+or GPC+RNA+viral particles. Reverse transcriptase RT-qPCR with primers targeting the short (e) or the large (f) segment of JUNV is shown. Error bars are the mean±s.d. of triplicates. Figure 4: Correlation between GPC levels and RNA content. FVA of JUNV particles stained with Alexa 647 GPC antibody only ( a ) or YOYO-1 only ( b ). Dot plots represent nucleic acid dye fluorescence ( x axis) as a function of the Alexa 647 GPC fluorescence ( y axis). ( c ) Flow virometry analysis of particles stained with both Alexa 647 GPC antibody and the nucleic acid dye YOYO-1. ( d ) Pie charts representing the percentage of total RNA+ vesicles (green) and the percentage of potentially infectious particles (GPC + RNA + ; yellow) in the low and high fractions. The high fraction contains about 2.5 times more virions with both genetic material and surface GPC than the low fraction. ( e , f ) Relative amount of RNA contained in 20,000 sorted particles from total RNA + or GPC + RNA + viral particles. Reverse transcriptase RT-qPCR with primers targeting the short ( e ) or the large ( f ) segment of JUNV is shown. Error bars are the mean±s.d. of triplicates. Full size image Role of cholesterol-enriched membranes in JUNV infectivity Since FVA enables us to define specific virion's properties, we next investigated how the cholesterol content at the plasma membrane influences JUNV budding and infectivity. Cholesterol is an important component of cellular membranes that favours protein cluster microdomains by rigidifying lipid bilayers and could therefore influence GPC and cellular components incorporation into viral particles. We first examined the viral particle surface distributions of the Tetraspanin CD9, marker of the Tetraspanin-enriched microdomains (TEM) and the CTB, which binds to GM1 gangliosides and localizes primarily to lipid rafts. Both of these plasma membrane subdomains are enriched in cholesterol [19] , [20] . FVA analysis of JUNV-A647 particles co-stained with either an anti-CD9 antibody conjugated to Phycoerythrin (CD9-PE) or a CTB recombinant protein coupled to fluorescein isothiocyanate revealed that JUNV particles contain high levels of CD9 and CTB ( Fig. 5a,b ). Single staining controls showed no crosstalk between fluorophores ( Supplementary Fig. 4a,b ). Immunofluorescence and confocal spinning disk microscopy of JUNV-A647 particles spread on glass and stained with CD9-PE antibody confirm that CD9 is indeed enriched at the surface of JUNV particles ( Fig. 5c ; Pearson correlation coefficient: 0.77±0.1). Moreover, staining of infected cells with GPC and CD9 antibodies also illustrate that clusters of GPC at the plasma membrane are found in CD9-enriched regions (pink arrows in Fig. 5d ). These results further suggest that virions bud at specialized regions of the plasma membrane. 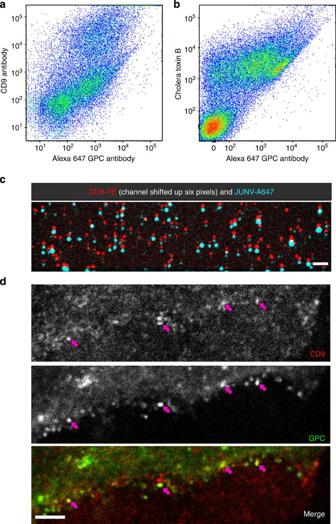Figure 5: JUNV buds at CD9-enriched sites. JUNV-A647 viral particles stained with either a CD9 antibody conjugated to PE (a) or CTB conjugated to FITC (b) were analysed by flow virometry and plotted as a function of Alexa 647 GPC antibody staining. (c) JUNV particles stained with a GPC antibody coupled to an Alexa Fluor 647 as inFig. 1g, were adsorbed on glow-discharged glass coverslip. Samples were blocked in 0.5% BSA in PBS for 30 min, incubated with mouse anti-CD9 antibody coupled to PE for 30 min and then washed extensively in 0.5% BSA in PBS. Coverslips were mounted on slides and imaged by spinning disk confocal microscopy. The micrograph represents CD9-PE (red) and JUNV-A647 (cyan) and the red channel was shifted by six pixels up to better appreciate colocalization of the two fluorophores. Over 500 JUNV-A647 particles were counted and Pearson correlation with CD9-PE was evaluated at 0.77±0.1. Scale bar, 5 μm. (d) Vero cells infected with JUNV for 24 h were fixed, permeabilized and stained with a CD9 antibody conjugated to PE and the GPC-specific GD01 antibody conjugated to Alexa Fluor 488. Images were acquired by spinning disk confocal microscopy and represent the plasma membrane of an infected cell. The images show CD9 staining (upper panel), GPC staining (middle panel) and the overlay of the two channels (bottom panel). The pink arrows highlight GPC positive spots, likely corresponding to budding events that are enriched in CD9. Scale bar, 5 μm. Figure 5: JUNV buds at CD9-enriched sites. JUNV-A647 viral particles stained with either a CD9 antibody conjugated to PE ( a ) or CTB conjugated to FITC ( b ) were analysed by flow virometry and plotted as a function of Alexa 647 GPC antibody staining. ( c ) JUNV particles stained with a GPC antibody coupled to an Alexa Fluor 647 as in Fig. 1g , were adsorbed on glow-discharged glass coverslip. Samples were blocked in 0.5% BSA in PBS for 30 min, incubated with mouse anti-CD9 antibody coupled to PE for 30 min and then washed extensively in 0.5% BSA in PBS. Coverslips were mounted on slides and imaged by spinning disk confocal microscopy. The micrograph represents CD9-PE (red) and JUNV-A647 (cyan) and the red channel was shifted by six pixels up to better appreciate colocalization of the two fluorophores. Over 500 JUNV-A647 particles were counted and Pearson correlation with CD9-PE was evaluated at 0.77±0.1. Scale bar, 5 μm. ( d ) Vero cells infected with JUNV for 24 h were fixed, permeabilized and stained with a CD9 antibody conjugated to PE and the GPC-specific GD01 antibody conjugated to Alexa Fluor 488. Images were acquired by spinning disk confocal microscopy and represent the plasma membrane of an infected cell. The images show CD9 staining (upper panel), GPC staining (middle panel) and the overlay of the two channels (bottom panel). The pink arrows highlight GPC positive spots, likely corresponding to budding events that are enriched in CD9. Scale bar, 5 μm. Full size image To investigate the role of cholesterol in JUNV budding and infectivity, we next performed FVA on viruses treated with the cholesterol depletion agent Methyl-β-Cyclodextrin (MβCD). The organization of both TEMs and lipid rafts are perturbed by MβCD treatment [19] , [20] . Vero cells infected for 24 h with JUNV were treated for 1 h with 10 mM MβCD, followed by extensive washes and incubation for an additional 12 h. It has been previously shown that cholesterol extraction by MβCD treatment lasts at least 12 h (ref. 21 ). Harvested supernatant, containing virions produced during the 12 h incubation period in absence of cholesterol, was prepared as previously described in Fig. 1g and analysed by FVA. MβCD-treated virions showed a strong reduction in CD9 staining at their surface compared with mock-treated virions ( Fig. 6a,b ). We then used 8,000 sorted particles from each condition to infect Vero cells. After 16 h, cells were harvested, fixed, permeabilized and stained with an antibody raised against the nucleoprotein (NP) of the virus and coupled to an Alexa Fluor 647 to measure the percentage of infected cells by flow cytometry ( Fig. 6c ). Cells treated with MβCD produced virions that were significantly less infectious than their mock counterpart, suggesting that cholesterol depletion alters infectivity, potentially by interfering with GPC incorporation into viral particles. 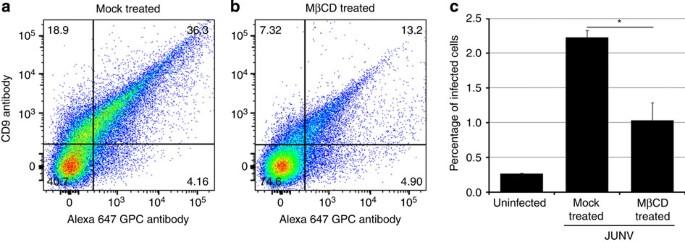Figure 6: Cholesterol depletion of producer cells decreases infectivity of budding viruses. Vero cells infected for 24 h with JUNV were mock treated (a) or treated with 10 mM Methyl-β-Cyclodextrin (MβCD-treated;b) for 1 h at 37 °C. Cells were then extensively washed with PBS and incubated for an additional 12 h at 37 °C. Subsequently, the supernatant was harvested and stained with LD05 GPC antibody conjugated to Alexa Fluor 647 and CD9 antibody conjugated to PE as inFig. 5a. Dot plots show CD9 antibody fluorescence as a function of Alexa 647 GPC antibody staining. Percentages in each corner indicate the proportion of each population in the given quadrant. The data shows that MβCD treatment strongly decreases CD9 at the surface of virions. (c) JUNV-A647 particles from MβCD or mock-treated producer cells were sorted and 8,000 particles per conditions were used to infect Vero cells for 16 h. Subsequently, the Vero cells were stained with a viral NP-specific antibody conjugated to an Alexa Fluor 647 and analysed by flow cytometry to measure the percentage of infected cells. A twofold decrease in infectivity was observed when producer cells were treated with MβCD compared to the mock condition. Error bars are the mean±s.d. of duplicates where at least 10,000 cells per sample were acquired. The difference marked by the star is significant (unpairedt-testPvalue=0.024). Figure 6: Cholesterol depletion of producer cells decreases infectivity of budding viruses. Vero cells infected for 24 h with JUNV were mock treated ( a ) or treated with 10 mM Methyl-β-Cyclodextrin (MβCD-treated; b ) for 1 h at 37 °C. Cells were then extensively washed with PBS and incubated for an additional 12 h at 37 °C. Subsequently, the supernatant was harvested and stained with LD05 GPC antibody conjugated to Alexa Fluor 647 and CD9 antibody conjugated to PE as in Fig. 5a . Dot plots show CD9 antibody fluorescence as a function of Alexa 647 GPC antibody staining. Percentages in each corner indicate the proportion of each population in the given quadrant. The data shows that MβCD treatment strongly decreases CD9 at the surface of virions. ( c ) JUNV-A647 particles from MβCD or mock-treated producer cells were sorted and 8,000 particles per conditions were used to infect Vero cells for 16 h. Subsequently, the Vero cells were stained with a viral NP-specific antibody conjugated to an Alexa Fluor 647 and analysed by flow cytometry to measure the percentage of infected cells. A twofold decrease in infectivity was observed when producer cells were treated with MβCD compared to the mock condition. Error bars are the mean±s.d. of duplicates where at least 10,000 cells per sample were acquired. The difference marked by the star is significant (unpaired t -test P value=0.024). Full size image This decrease in infectivity could also be explained by a defect in budding, as we detected half as many GPC + particles by FVA in virions coming from MβCD-treated cells compared to virions produced by non-treated cells ( Fig. 6a,b ). To test this hypothesis, we used reverse transcription RT-qPCR to measure the viral RNA content of cells and supernatant in samples treated or not with MβCD as described in Fig. 6 , normalized to the housekeeping gene glyceraldehyde 3-phosphate dehydrogenase. The amounts of short and large RNA segments in cells and supernatant were unaffected on MβCD treatment ( Supplementary Fig. 5a,b ), suggesting that cholesterol depletion does not affect JUNV budding and release. Thus, the observed decrease in GPC positive particle detection by FVA could be attributed to low GPC incorporation resulting in an inability to reach the threshold of detection of our cytometer. In conclusion, the concentration of GPC at the virion surface and potentially other cellular factors such as CD9 enrichment could be key factors to enhance viral infectivity. Our study presents the first successful attempt to use high-resolution flow cytometry to analyse and sort small lipid vesicles, while preserving their biological activity, using the JUNV as a model system. This method allows us to characterize the molecular pattern of viral particles and highlights that Junin virions are heterogeneous in morphology and nature, which influences their infectivity capacities. We have used high-powered lasers and enhanced optics combined with a new variable DFS to improve the resolution and sensitivity of our cytometer. We have been able to detect 40 nm fluorescent beads and also to sort 50–60 nm enveloped viral particles by flow virometry using a combination of forward scatter and fluorescence intensities ( Fig. 1 ). Previously, a few groups have been able to analyse small vesicles using flow cytometry [2] , [3] , [4] , [5] , [6] , [7] , [8] . However, to our knowledge, the study by Allen et al . [8] is the only one that succeeded to sort bacteriophages (of about 200 nm in length) for further genome sequencing, although no functional biological assay post sort could be performed. Differentiation of single and multiple events, when analysing cells by flow cytometry, is usually based on multiple forward scatter angles such as FSC-A, FSC-H or FSC-W parameters. In the case of small vesicles, it becomes technically challenging to prove that each sorting droplet contains a single viral particle. A previous study that attempted small particle sorting used a large 140 μm nozzle and a sheath pressure of 5 p.s.i. [3] but the authors suggested that using a smaller nozzle size and higher pressure would improve the sorting of nanosized vesicles. In agreement with this study, we found that a 70 μm nozzle and a high flow pressure of 70 p.s.i. (482 kPa) results in a smaller drop size and therefore, statistically reduces the probability of sorting several events in a single droplet. Yet, further technological advances are required to prove in a more direct manner that each individual droplet contains a single particle. The size of particles present in different populations has been difficult to accurately determine by direct comparison with beads, as correlation between actual bead size and instrument light scatter measurements varies according to the specific refractive index of the particles analysed [17] . The most accurate way to measure the size of particles remains EM. Using EM, we observed a clear difference between the low and high fractions obtained from FVA, with sizes around 60 and 150 nm, respectively. Moreover, we used TSRP to further analyse the sorted particles and confirmed that FVA allows sorting of particles smaller than 300 nm ( Fig. 2c ). In the future, coupling FVA to other advanced techniques of cytometry such as Pulse Shape Analysis [22] , [23] , could further improve the resolution and may provide single molecule sensitivity as is currently achieved for techniques such as total internal reflection fluorescence microscopy [24] . We used FVA to analyse JUNV particles and discovered several interesting features. First, we observed that two viral populations of different sizes co-exist, though size heterogeneity is usually unexpected for small RNA viruses. Interestingly, a recent study investigating the protein composition of hundreds of single HIV virions using optical tweezers and super-resolution microscopy highlighted that HIV particles are also very heterogeneous in size and in the amount of viral envelope proteins they exhibit on their surface [25] . Viruses use envelope GPCs for the initial recognition of their cellular receptor at the surface of target cells. Such interactions are indispensable for efficient entry, infection and subsequent spreading to other cells. However, the amount of envelope proteins at the surface of a particle and the number of envelope proteins actually required to facilitate efficient cell entry is variable according to the virus family (for examples, see refs 26 , 27 , 28 ). The amount of GPC incorporated by a given virus particle may be critical to establish its infectivity potential and FVA could represent a powerful tool to study the amount of receptors potentially engaged, as it has been previously investigated by light microscopy [24] . Future investigations will benefit from newly developed high-resolution cytometers and microscopes to identify additional factors present at the virion surface that influence their infectivity. In our study, we hypothesized that the difference in infectivity between populations could be attributed to the virion RNA content, as JUNV possesses two segments in its genome, and therefore, small particles may encapsidate only one of the two segments. This hypothesis was ruled out by RT-qPCR experiments that demonstrated similar RNA amounts and short/large segment ratios between the low and high fractions ( Fig. 3 ). Moreover, while GPC + RNA + particles were 2.5 times enriched in the high fraction compared with the low one, both fractions contained comparable percentages of total RNA + particles ( Fig. 4d ). These results indicate that the low fraction may contain more ‘naked’ particles (RNA + GPC − ) than the high fraction. It is considered that the type of producer cell may affect the nature of released viruses. However, using conventional virology assays, it is intricate to correlate and control for particle size, infectivity and RNA content as a function of the cell type from which they were produced. FVA allowed us to compare the infectivity of JUNV particles produced by physiologically relevant macrophages [29] , [30] to those produced by Vero cells. We found that JUNV particles produced by macrophages were poorly infectious compared with those produced by Vero cells ( Fig. 3e ). This may be explained by the fact that Vero cells lack a functional interferon-α/β response and exhibit poor immune capacities, while macrophages are highly potent immune cells and may therefore have intrinsic mechanisms that prevent proper JUNV assembly. In the future, FVA could be further developed to determine what these mechanisms are, by investigating the role of cytokines and intracellular immune sensors during viral assembly/release. We found that JUNV particles bud at specialized lipid membrane microdomains and disruption of these domains by cholesterol depletion decreases JUNV infectivity ( Figs 5 and 6 ). It has recently been shown that JUNV GPC associates primarily with lipid raft cholesterol-enriched membranes and that cholesterol extraction decreases GPC association with the cell membrane [31] . In contrast, Agnihothram et al . [32] reported that GPC localizes to soluble lipid microdomains distinct from conventional lipid rafts. These two studies mainly utilized biochemical techniques to define GPC location. By FVA and confocal microscopy, we now show that JUNV particles are CD9 (TEM marker) and CTB (gold standard lipid raft marker) positive. Of note, HIV induces the coalescence of lipid raft and TEM [33] and one possibility is that JUNV operates similarly during budding, which would explain why both CD9 and CTB are found on viral particles. On cholesterol depletion, we observed by RT-qPCR that the same amount of viral RNA was produced by and secreted from JUNV infected cells ( Supplementary Fig. 5 ) but that fewer GPC positive virions were detected by FVA ( Fig. 6a,b ). This could be due to the cells releasing more ‘naked’ viruses that do not have detectable levels of GPC at their surface. Depletion of cholesterol from the plasma membrane may also lead to a decreased viral particle incorporation of specific cellular lipids and proteins that are important for attachment/entry steps and thus, infectivity. Further work is required to define how cellular lipids and proteins impact virion infectiveness. CD9 is also considered a protein marker for extracellular vesicles [34] , [35] , while CTB is an emerging marker for lipid raft [36] , [37] , [38] . In our FVA experiments, a subset of virus particles negative for GPC were CTB positive, indicating that our viral preparation also contained microvesicles that were efficiently discriminated from ‘true’ viral particles ( Fig. 5b ). In contrast, most CD9 + events were associated with viral particles ( Fig. 5a ), suggesting that subpopulations of cellular lipid microvesicles co-exist in our viral preparations, and that FVA has the potential to differentiate between populations. In conclusion, we have developed a new analytical approach to quantitatively study large numbers of functional virions in an efficient and reliable manner. The ability to resolve and sort functional subsets of nanosized lipid vesicles has broad applications in various fields. Our FVA can be applied to many virus families as well as different types of intra/extracellular vesicles. Virus maintenance Vero cells (ATCC) were maintained at 37 °C and 5% CO 2 in Dulbecco’s Modified Eagle’s medium (DMEM) media (Life Technologies-Gibco) supplemented with 10% heat inactivated fetal bovine serum (FBS; Atlanta Biologicals), 100 IU ml −1 penicillin and 100 mg ml −1 streptomycin and 2 mM L -Glutamine (Life Technologies-Gibco). Within the text, Junin virus or JUNV refers to the non-pathogenic vaccine strain Candid1 (obtained from the Bavari laboratory at USAMRID), which is the only strain used in this study. JUNV production was performed by inoculation of JUNV (passage 2) to subconfluent Vero cells at a multiplicity of infection of 0.5 in a low volume of Virus media: DMEM (Life Technologies-Gibco) supplemented with 2% heat inactivated FBS (Atlanta Biologicals), 100 IU ml −1 penicillin and 100 mg ml −1 streptomycin and 2 mM L -Glutamine (Life Technologies-Gibco). After 1 h, additional media was provided and cells were incubated for 72 h at 37 °C, 5% CO 2 . Supernatant was harvested and cleared from cellular debris by centrifugation at 10,000 g at 4 °C for 10 min. The virus-containing supernatant was then frozen at −80 °C before use. Viruses were titrated by plaque assay on Vero cells. Virus labelling JUNV stock was incubated with a non-neutralizing mouse monoclonal antibody raised against the JUNV Envelope GPC (4 μg ml −1 ; LD05-BF09; NR-2569; BEI resources), coupled to an Alexa Fluor 647 for 30 min at 25 °C. Viruses were also labelled with YOYO-1 (100 nM; Life Technologies), CD9 monoclonal antibody conjugated to Phycoerythrin (PE; 1 μg ml −1 ; BD Biosciences) or CTB conjugated to fluorescein isothiocyanate (FITC; 4 μg ml −1 ; Sigma-Aldrich) according to the experiment. The virus-dye mixture was then gently applied on top of a 10% Optiprep (Sigma-Aldrich) cushion and ultracentrifuged at 150,000 g for 2 h at 4 °C using rotor SW55 Ti (Beckman Coulter). The supernatant was discarded and pellets were resuspended in 0.2 μm filtered PBS, 1% bovine serum albumin (BSA) and left overnight in the dark at 4 °C for gentle solubilization. The preparation was used the next day for FVAs. Monocyte-derived macrophages Blood of healthy donors was obtained from the Kraft Family Blood Donor Center (informed consent signed by the donors). Peripheral blood mononuclear cells were isolated by Ficoll (GE Healthcare). Monocytes were purified by positive selection using CD14+ Microbeads (Miltenyi) and differentiated into macrophages for 7 days in RPMI (Life Technologies-Gibco) supplemented with 10% FBS, heat inactivated at 56 °C, Premium select triple 0.1 μm filtered (FBS; Atlanta Biologicals), 100 IU ml −1 penicillin and 100 mg ml −1 streptomycin, 2 mM L -Glutamine (Life Technologies-Gibco) and supplemented with 25 ng ml −1 macrophage colony-stimulating factor as in ref. 39 . RNA analysis Total RNA from cells was purified using the RNeasy Mini kit (Qiagen). Reverse transcription and RT-qPCR amplifications were performed using the one step QuantiFast SYBR Green RT-PCR kit (Qiagen). Viral and cellular DNAs were detected using specific primers for the short segment (5′- cctagcgcttgcaggaagatcc -3′ and 5′- caccagctcatatctgctggatg -3′), the large segment (5′- ggagggtagctcacagcagtc -3′ and 5′- ctatggtggtggtgctgttggc -3′) and the glyceraldehyde 3-phosphate dehydrogenase (5′- gagtcaacggatttggtcgt -3′ and 5′- ttgattttggagggatctcg -3′). The amplification conditions were as follow: reverse transcription, 10 min at 50 °C; PCR initial activation step, 5 min at 95 °C; 40 cycles of denaturation and combined annealing/extension, 10 s at 95 °C and 30 s at 60 °C, respectively. Fluorescence data collection was acquired at the end of each cycle, and a melting curve showing specificity of the primers used was included at the end of each PCR reaction. FVA and sorting A 15-channel FACSAria II Special Order (SORP) cell sorter cytometer (BD Biosciences) equipped with a combination of 355, 407, 488, 640 and 594 nm lasers was used. Fluorescence emission was collected through 530/30 (FITC), 575/25 (PE) and 660/20 (Alexa 647) bandpass filters. The instrument was upgraded with a high-powered 488 nm, 300 mW (263 mW at the stream) special order laser (Coherent Inc), a variable DFS option and laser tunable software, Coherent Connection (Coherent Inc.). The forward scatter includes a high-sensitivity photomultiplier tube (FSC-PMT) and improved collection optics, allowing the detection of nanosized microvesicles and viral particles [5] , [6] . Fluid sheath running through the cytometer was highly filtered (0.45 and 0.1 μM filters). Sorting was performed with a 70 μm nozzle, a pressure of 70 p.s.i. (482 kPa) and frequency of 87,500. The droplet size was experimentally measured to be 1.5 to 1.7 nl. Preliminary set-up and alignment of the FSC-PMT-A was performed using a set of polystyrene size beads (300, 500, 800 nm; BD Biosciences) and fluorochrome-conjugated carboxylated-modified latex beads (40 nm APC-conjugated and 100 nm PE-conjugated beads; Life Technologies). The DFS consists of a tunable picomotor-driven device that allows accurate adjustment of the laser beam size at the core of the stream, therefore increasing the scatter signal and decreasing the background. Before start experiments, the DFS optimal parameters were determined on dedicated BD software using Megamix Plus-FSC beads (BioCytex). All data were analysed using FACSDiva 6.1 (BD Biosciences) and FlowJo 10.0.7 (Treestar Inc.) software. Tunable resistive pulse sensing JUNV-A647 preparation resuspended in filtered PBS was sorted or not and then applied on a qViro-X system (IZON Science) as described in ref. 18 . In brief, 40 μl of the viral preparation in ultra-filtered PBS was added on top of a thermoplastic polyurethane membrane with a single nanopore (NP150) at 46.87 mm stretch, 0.70 V and 1.2 KPa of applied pressure. The ionic current and resistive pulse signals were collected using IZON proprietary software. The measurement was calibrated using 115 nm polystyrene calibration beads (Bangs Laboratories). Virus infectivity assays Infectivity of JUNV was measured by plaque assay or by flow cytometry. For plaque assay, confluent Vero cells were inoculated with serial dilution of JUNV for 1 h at 37 °C. Cells were then covered with an overlay composed of 1% agarose diluted in Virus media. Five days post infection, cells were fixed with 10% formaldehyde for 30 min. The overlay was then discarded and the cell monolayer was stained with 0.05% crystal violet in 10% ethanol. Plaques were counted in the well containing the appropriate virus dilution. For flow cytometry, Vero cells were infected with particles sorted by FVA. After 16 h, cells were harvested, fixed with 4% paraformaldehyde and permeabilized with 0.5% BSA and 0.05% saponin in PBS, followed by incubation with a mouse monoclonal antibody (2 μg ml −1 ; SA02-BG12; NR-2573; BEI resources) specific for the JUNV NP and coupled to an Alexa Fluor 647. Acquisition of fluorescence intensity of the infected cells was performed on a FACSCanto II with 488 and 640 nm lasers (BD Biosciences). Analysis of the percentage of infected cells was completed using FlowJo version 10.0.7 (Treestar Inc). Immunofluorescence and light microscopy Infected Vero cells were fixed, permeabilized with 0.5% BSA and 0.05% saponin in PBS and co-stained with a mouse monoclonal antibody (4 μg ml −1 ; GD01-AG02; NR-2565; BEI resources) specific for the JUNV GPC and conjugated to an Alexa Fluor 488 and the CD9 monoclonal antibody conjugated to PE (2 μg ml −1 ; BD Biosciences). The samples were imaged on a Zeiss AxioObserver.Z1 inverted microscope mounted with a spinning disc head (Yokogawa), a QuantEM:512SC EMCCD camera (Photometrics) and a × 100, 1.4 NA oil objective (Zeiss). Transmission electron microscopy Low and high fractions were sorted directly on glow-discharged carbon-coated EM grids (Electron Microscopy Sciences). Samples were then incubated with the uncoupled mouse monoclonal antibody raised against GPC (10 μg ml −1 ; GD01-AG02; NR-2565; BEI resources), followed by a secondary Rabbit anti-mouse antibody (MP Biomedicals) and revealed by Protein A conjugated to 10 nm gold beads. Negative staining was achieved by incubating samples in Uranyl formate (Electron Microscopy Sciences) for 30 s. The grids were examined on a JEOL 1200EX Transmission electron microscope and images were recorded with an AMT 2k CCD. How to cite this article: Gaudin, R. & Barteneva, N.S. Sorting of small infectious virus particles by flow virometry reveals distinct infectivity profiles. Nat. Commun. 6:6022 doi: 10.1038/ncomms7022 (2015).